Unique features of mutations revealed by sequentially reprogrammed induced pluripotent stem cells Although viable mice can be generated from induced pluripotent stem cells (iPSCs), the impact of accumulated mutations on the developmental potential of the resulting iPSCs remains to be determined. Here, we demonstrate that all-iPSC mice generated through tetraploid blastocysts complementation can tolerate the accumulation of somatic mutations for up to six generations using a Tet-on inducible reprogramming system. But, the viability of the all-iPS mice decreased with increasing generations. A whole-genome sequencing survey revealed that thousands of single-nucleotide variations (SNVs), including 44 non-synonymous ones, accumulated throughout the sequential reprogramming process. Subsequent analysis provides evidence that these accumulated SNVs account for the gradual reduction in viability of the resultant all-iPSC mice. Unexpectedly, our present reprogramming system revealed that pluripotent stem cells are heterogeneous in terms of possessing a set of copy-number alterations (CNAs). These CNAs are unique for pluripotent cells and subsequently disappear in the differentiating progenies. The successful reprogramming of differentiated somatic cells into pluripotent stem cells has revolutionized our understanding of cell plasticity [1] , [2] . The generation of patient-specific pluripotent stem cells directly from somatic cells has raised the possibility of utilizing these personalized pluripotent stem cells in regenerative medicine, pathological studies and drug screening [3] , [4] , [5] , [6] . Somatic cell nuclear transfer (SCNT) and the induction of pluripotency by defined transcription factors are two major approaches that can reprogram differentiated mammalian somatic cells to a pluripotent and even a totipotent state by SCNT [1] , [2] , [7] , [8] , [9] , [10] , [11] . The results of a very recent study have demonstrated that mice can be successfully re-cloned to more than 25 generations through serial nuclear transfer, which indicates that a very strict selection strategy to eliminate the defective cloned embryos during development might be utilized in SCNT-mediated reprogramming [12] . Similarly, we and others have previously shown that induced pluripotent stem cells (iPSCs) reprogrammed via a Tet-on inducible reprogramming system can also produce all-iPSC clonal mice through tetraploid blastocyst complementation [13] , [14] , [15] , [16] . However, the number of generations of all-iPSC mice that can be serially produced using this inducible iPS system has not been determined. It has been reported that defined transcription factors that mediate reprogramming can potentially induce or enlarge mutations in the resultant iPSCs, but the impact of the mutations on the developmental potential of resultant iPSCs remains to be evaluated [17] , [18] , [19] , [20] , [21] . The Tet-on inducible iPS system provides an invaluable framework that enables the evaluation of the developmental potential of sequentially reprogrammed iPSCs and the determination of the effects of genetic alterations. Here, we demonstrate that the accumulation of somatic mutations was tolerated by all-iPSC mice for up to six generations, but directly impacted the survival of all-iPSC mice in later generations. Generation of adult all-iPSC mice to three generations Using a sequential reprogramming approach based on the doxycycline (Dox)-inducible iPS system, we first aimed to determine whether viable all-iPSC mice with normal fertility could be sequentially produced through tetraploid blastocyst complementation in a similar manner to that used to produce serial cloned mice through somatic cell nuclear transfer (SCNT) [22] ( Fig. 1a ). The 1 0 -all-iPSC mice were generated from one Tet-on inducible iPSC line that was initially derived from mouse embryonic fibroblasts (MEFs) with the 129/Sv × M2rtTA genetic background [23] . Subsequently, adipocyte progenitor cells (APCs) were retrieved from the adipose tissue of the 1 0 -all-iPSC mice ( Supplementary Fig. 1a,b ). After the addition of Dox to the induction medium, 2 0 -iPSC colonies emerged that exhibited the typical ESC-like morphology and positive staining for alkaline phosphatase (AP) ( Supplementary Fig. 1c,d ). After propagation, pluripotency markers, including Oct4 (also known as Pou5f1), Nanog, Sox2 and the ESC-specific surface marker SSEA-1, were positively expressed in the 2 0 -iPSCs ( Supplementary Fig. 1e ). Bisulfite genomic sequencing analysis of the DNA methylation status of the Pou5f1 and Nanog promoters confirmed that DNA demethylation had occurred during secondary reprogramming ( Supplementary Fig. 1f,g ). The silencing of the exogenous factors was further confirmed in the iPSC lines that were tested ( Supplementary Fig. 1h ). Furthermore, after the injection of iPSCs into severe combined immunodeficient mice, the formation of teratomas with three germ layers was observed ( Supplementary Fig. 1i ). Moreover, chimeric mice (2 N) with germline transmission ability could be produced from these 2 0 -iPSC lines ( Supplementary Fig. 1j ). Most importantly, viable fertile all-iPSC mice could be generated from the APC-derived 2 0 -iPSC lines through tetraploid complementation ( Fig. 1b ). Subsequently, we produced a third generation of viable all-iPSC mice with normal fertility from the 3 0 -iPSC lines that were established from APCs retrieved from the 2 0 -all-iPSC mice ( Fig. 1b ). Simple sequence length polymorphism (SSLP) analyses were performed, which confirmed that the all-iPSC mice were indeed produced from iPSCs ( Fig. 1c ). We concluded that adult all-iPSC mice with normal fertility could be produced using this Tet-on inducible iPS system. 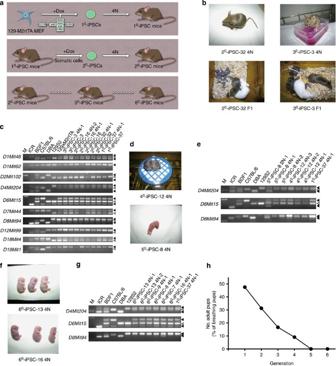Figure 1: Sequentially reprogrammed iPSCs support the production of all-iPSC mice for up to six generations. (a) A schematic diagram for the production of all-iPSC mice for up to six generations using sequentially reprogrammed iPSCs. (b) The viable all-iPSC mice that were derived from sequentially reprogrammed iPSC lines (20-iPSCs and 30-iPSCs) through tetraploid complementation (top) and the offspring (F1) of the all-iPSC mice (bottom). (c) SSLP analysis for the genetic identification of the all-iPSC mice. (d,e) The all-iPSC mice derived from 40-iPSC, 50-iPSC (d) and SSLP analysis for the genetic identification of all-iPSC mice (e). (f,g) The all-iPSC mice derived from 60-iPSC (f) and SSLP analysis for the genetic identification of all-iPSC mice (g). (h) The percentage of live-born all-iPSC pups that reached adulthood in each generation. Figure 1: Sequentially reprogrammed iPSCs support the production of all-iPSC mice for up to six generations. ( a ) A schematic diagram for the production of all-iPSC mice for up to six generations using sequentially reprogrammed iPSCs. ( b ) The viable all-iPSC mice that were derived from sequentially reprogrammed iPSC lines (2 0 -iPSCs and 3 0 -iPSCs) through tetraploid complementation (top) and the offspring (F1) of the all-iPSC mice (bottom). ( c ) SSLP analysis for the genetic identification of the all-iPSC mice. ( d , e ) The all-iPSC mice derived from 4 0 -iPSC, 5 0 -iPSC ( d ) and SSLP analysis for the genetic identification of all-iPSC mice ( e ). ( f , g ) The all-iPSC mice derived from 6 0 -iPSC ( f ) and SSLP analysis for the genetic identification of all-iPSC mice ( g ). ( h ) The percentage of live-born all-iPSC pups that reached adulthood in each generation. Full size image Reduced viability of all-iPSC mice with increasing generations To further ascertain whether viable adult all-iPSC mice with normal fertility could be generated to many generations, we established 4 0 -, 5 0 - and 6 0 -iPSC lines from the somatic cells retrieved from the previous generations of all-iPSC mice, and 4 0 -, 5 0 - and 6 0 -all-iPSC mice were subsequently produced through tetraploid complementation ( Fig. 1d–g ). In summary, the average induction efficiency of sequential reprogramming based on AP staining was ~0.7% ( Supplementary Fig. 1k ), and the efficiency of all-iPSC mouse formation (average 1.4%) was comparable to that described in recent reports [14] ( Supplementary Table 1 ). However, the viability of the all-iPSC mice produced was greatly reduced with increasing generations. For example, the 1 0 –3 0 -all-iPSC mice could grow into fertile adults, while the 4 0 -all-iPSC and 5 0 -all-iPSC mice only survived up to 4 weeks and 2 days, respectively. Most strikingly, all of the 27 6 0 -all-iPSC mice died immediately after caesarean section ( Fig. 1h and Supplementary Table 1 ). We first performed 5-methylcytosine (5-mC) MeDIP-seq and RNA-seq analysis of the sequentially reprogrammed iPSC lines. The results revealed that only a few differential methylation regions (DMRs) located in gene promoter regions displayed an accumulating pattern. However, the expression traces in sequentially reprogrammed iPSC of downstream genes demonstrated that no genes were cis-regulated by an accumulating pattern of differential methylation in the promoter region ( Supplementary Fig. 2 ). Moreover, in a recent study, we have demonstrated that the core histone modifications (H3K4me2, H3K4me3, H3K27me3) are comparable among iPSC lines that can produce all-iPSC mice [24] . Taken together, we conclude that although all-iPSC mice can be produced up to six generations, their viability decreases with increasing generations, and epigenetic effects might not be a major cause of this reduction in viability. Single-nucleotide variations accumulated during sequential reprogramming To further investigate whether sequential reprogramming altered the genome integrity of the resultant iPSCs and subsequently affected the viability of all-iPSC mice, a whole-genome sequencing approach was applied to investigate the effects of genetic alterations on the developmental potential of the sequentially reprogrammed iPSCs. DNA was extracted from a total of eight sequentially reprogrammed iPSC lines and five parental somatic cells. Paired-end reads of up to 150 Giga and 50 × for the mouse genome were generated for each sample using a Hiseq 2000 sequencer ( Supplementary Fig. 3a ). The paired-end reads and gene expression analyses confirmed that there were nine stable lentiviral integration sites in the exogenous Oct4, Sox2, Klf4 and c-Myc vectors in the genomes throughout the sequential reprogramming process, and these sites did not disrupt any endogenous genes ( Supplementary Fig. 3b and Supplementary Data 1 ). Thousands of single-nucleotide variations (SNVs) that occurred throughout the sequential iPS process were surveyed by pair-wise comparisons among the samples. The SNVs were fractionated according to the various accumulating patterns ( Fig. 2a and Supplementary Fig. 3c ). A total of 189 SNVs, including all of the coding SNVs, were verified via Sequenom genotyping in all 13 samples in addition to the feeder cell line ( Supplementary Fig. 3d,e and Supplementary Data 2 ). The genotyping results also suggested that pollution of the feeder cells in the DNA isolation from the iPSC lines caused the recurrence of some SNVs in all of the iPSC lines ( Supplementary Data 2 ). 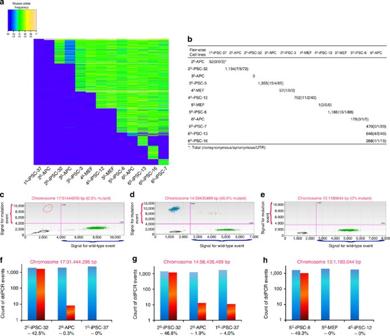Figure 2: The accumulated SNVs and their frequencies during sequential reprogramming. (a) A heat map of the dynamic frequencies representative of the type of accumulated SNVs on the trace of the sequential iPS procedures. Note: The DNA of the 30-APCs was extracted from three all-iPSC mice that were derived from the same iPSC line. (b) The numbers of accumulated SNVs emerged in each stage throughout the sequential reprogramming. (c) Detection of low frequencies of SNVs in the 20-APC by droplet digital PCR. The signal intensities associated with the PCR amplification across the mutant allele (yaxis, red) and the reference allele (xaxis, blue). The scatter dot surrounded by a red dashed circle represents the mutant allele. There were significantly fewer dots for PCR events in the SNV than in the reference allele. (d,e) A scatter plot showing the fixed accumulated SNVs confirmed in 60-iPSC-13 (d); the SNVs were not detected in 50-MEF somatic cells of the parental generation (e). (f) Droplet digital PCR analysis of an SNV showing that the accumulated SNV pre-existed in the somatic cells of the parental generation at low frequencies and reached high frequencies in subsequent iPSCs. Counts of ddPCR events for SNVs (blue bar) and the reference (red bar) resulted in an estimated cell frequency in 20-iPSC-32, 20-APC, and 10-iPSC-37 of 42.5%, 0.3%, 0%, respectively. (g) The accumulated SNV pre-existed in somatic cells of the parental generation and previous iPS cell lines at a low frequency as detected by ddPCR analysis. (h) Droplet digital PCR analysis showing that the accumulated SNV was not detectable in the somatic cells of the parental generation and was detected in subsequent iPSCs with a relatively high frequency. Figure 2: The accumulated SNVs and their frequencies during sequential reprogramming. ( a ) A heat map of the dynamic frequencies representative of the type of accumulated SNVs on the trace of the sequential iPS procedures. Note: The DNA of the 3 0 -APCs was extracted from three all-iPSC mice that were derived from the same iPSC line. ( b ) The numbers of accumulated SNVs emerged in each stage throughout the sequential reprogramming. ( c ) Detection of low frequencies of SNVs in the 2 0 -APC by droplet digital PCR. The signal intensities associated with the PCR amplification across the mutant allele ( y axis, red) and the reference allele ( x axis, blue). The scatter dot surrounded by a red dashed circle represents the mutant allele. There were significantly fewer dots for PCR events in the SNV than in the reference allele. ( d , e ) A scatter plot showing the fixed accumulated SNVs confirmed in 6 0 -iPSC-13 ( d ); the SNVs were not detected in 5 0 -MEF somatic cells of the parental generation ( e ). ( f ) Droplet digital PCR analysis of an SNV showing that the accumulated SNV pre-existed in the somatic cells of the parental generation at low frequencies and reached high frequencies in subsequent iPSCs. Counts of ddPCR events for SNVs (blue bar) and the reference (red bar) resulted in an estimated cell frequency in 2 0 -iPSC-32, 2 0 -APC, and 1 0 -iPSC-37 of 42.5%, 0.3%, 0%, respectively. ( g ) The accumulated SNV pre-existed in somatic cells of the parental generation and previous iPS cell lines at a low frequency as detected by ddPCR analysis. ( h ) Droplet digital PCR analysis showing that the accumulated SNV was not detectable in the somatic cells of the parental generation and was detected in subsequent iPSCs with a relatively high frequency. Full size image The reduction in viability of the sequential all-iPSC mice demonstrated the impact of one type of SNV on the developmental potential of the resultant sequentially reprogrammed iPSCs. This SNV accumulated in each generation and then was inherited and fixed in subsequent offspring due to the induction of a genetic bottleneck. The heat map of the frequencies illustrated a dynamic trace of the accumulation of these SNVs, which were confirmed to have a high validation rate ( Fig. 2a ). The SNVs were subdivided according to the time of emergence across the sequential reprogramming, and then their numbers were calculated ( Fig. 2b ). Fifty-nine validated coding SNVs, including 44 non-synonymous SNVs, accumulated throughout the sequential process ( Table 1 ). Among them, 16 were annotated in the genes with lethal homozygous phenotypes in the Mouse Genome Informatics database ( Supplementary Table 2 ) [25] . In addition, on the basis of a survey of the literature, seven that accumulated during a later period of the sequential reprogramming were involved in genes with some heterozygous phenotypes ( Supplementary Table 2 ) [26] , [27] , [28] , [29] , [30] , [31] , [32] , [33] , [34] , [35] , [36] , [37] , [38] , [39] , [40] , [41] , [42] , [43] , [44] , [45] , [46] . In particular, Ep300 in 3 0 -iPSCs and subsequently Ryr2 in 5 0 -iPSCs shared similar one-allele mutant and haploinsufficiency phenotypes that were associated with cardiac developmental defect. In addition, mice with haploinsufficiency for Cd2ap exhibited a phenotype similar to human focal segmental glomerulosclerosis ( Supplementary Table 2 ). These phenotypes were supported by our histopathological examination of 6 0 -all-iPSC mouse tissues, which revealed an abnormal morphogenesis of the heart and kidney ( Supplementary Fig. 4 ). The combined effect of missense mutations in Ep300 , Ryr2 and Cd2ap might gradually disrupt the tolerable genetic load and account for the developmental failure of all-iPSC mice in late generations. Table 1 Comprehensive information about the SNVs located in the coding sequence (CDS) regions. Full size table Tracking causes of the accumulated single-nucleotide variations To distinguish the origins of these accumulated SNVs, we subsequently applied droplet digital PCR (ddPCR) to monitor the frequencies of these SNVs in parental somatic cells and iPSCs of previous generations ( Fig. 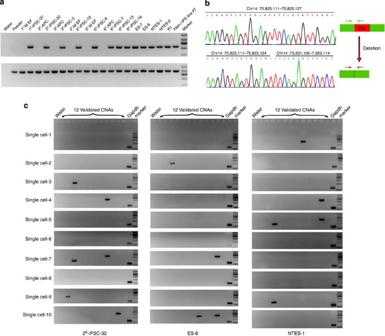Figure 3: Repeated copy-number alterations (CNAs) in pluripotent stem cells. (a) PCR results for the iPSC-specific CNA at chr14:75,825,104–75,831,195 (upper panel) and the control intact allele that retained the CNA (lower panel). A unique amplified breakpoint-spanning PCR product was present in all of the pluripotent stem cell lines but not in all of the somatic cell lines. (b) Sanger sequencing of the amplified band and schematic of the PCR validation assay design. The exact deletion breakpoints were confirmed, and the deleted regions were in accordance with the annotation of the retrotransposon (LINE). (c) The single-cell PCR results for all of the 12 validated CNAs (from lane 2 to lane 13 according to the chromosome position of the CNAs) in 20-iPSC-32, ES-8 and NTES-1. 2c–e and Supplementary Table 3 ) [47] , [48] . Three primary frequency patterns emerged of SNVs in iPSCs and are summarized in Fig. 2f–h . Two types of SNVs were pre-existing but distinct with regard to their time of origin. The first type of SNV with a fixed frequency in iPSCs had a low frequency only in the parental somatic cells ( Fig. 2f ), which occurred in cell divisions during the development of the all-iPSC mice. The second type exhibited a low frequency in both the parental somatic cells and the iPSCs of the early generations ( Fig. 2g ). Each SNV of the second type was initiated in an individual cell during cell culture of the early generations of the iPSC line but was retained in a mosaic all-iPSC mouse that was derived from the tetraploid complementation of the 10–15 iPSCs injection. The SNVs in the last category, which were considered de novo SNVs, had no detectable frequencies via ddPCR in parental somatic cells and iPSCs of the previous generation but were detected in subsequent iPSCs with a high frequency ( Fig. 2h ). 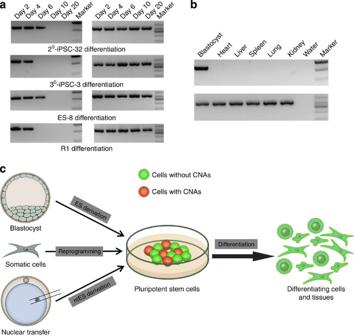Figure 4: Disappearance of CNAs during thein vitrodifferentiation of pluripotent stem cells and tissues. (a) PCR analysis of the gradually differentiated cells demonstrating that the validated CNA at chr14:75,825,104–75,831,195 became undetectable during thein vitrodifferentiation of iPSCs and ESCs (left image). The corresponding PCR results for the control are shown in the right image. (b) The CNA validated above could not be detected in all of the tested tissues but was detected in pre-implantation blastocysts by PCR (upper panel). A unique band retaining the LINE region was also produced by PCR (lower panel). (c) Summary model illustrating that the pluripotent stem cells were heterogeneous in terms of the repeated CNAs and that the CNAs were unique to pluripotent cells and subsequently disappeared in differentiating cells. In summary, at least two-thirds of the SNVs originated before iPSC induction and pre-existed in the all-iPSC mouse tissues ( Supplementary Table 4 ). Repeated CNAs observed in pluripotent stem cells Unlike SNVs, no apparent copy-number alterations (CNAs) accumulated during the sequential reprogramming. Instead, the genomic data for the sequential reprogramming revealed a pattern in which several uniform CNAs were found in each sequential iPSC lines but were not detected in the somatic cells derived from the all-iPSC mice. We excluded the pseudo-CNAs caused by replication timing, which could result in a gain or a loss in the read-depth profiles of the iPSC lines ( Supplementary Fig. 5a–c ) [49] , [50] , [51] . The breakpoints of the CNAs surveyed from the paired-end reads and the subsequent PCR results for multiple breakpoints supported the repeated occurrences of the true CNAs in the iPSC lines but not in the somatic cells and feeder cells during the sequential reprogramming ( Fig. 3a , Supplementary Fig. 2b and Supplementary Figs 6a–12a , Supplementary Data 3 ). The extended analysis further revealed that these repeated CNAs were obtained not only in the sequential iPSC lines but also in other SCNT-derived ES (ntES) cell lines, normal fertilization-derived ESC lines and an iPSC line generated in another laboratory ( Fig. 3a , Supplementary Figs 6a–12a and Supplementary Data 3 ). Sanger sequencing of PCR products of breakpoints revealed that each deleted fragment caused by the verified CNA included an annotation of a retrotransposon element, such as long interspersed nucleotide elements (LINEs) and long terminal repeats (LTRs) ( Fig. 3b and Supplementary Figs 6b–12b and Supplementary Data 3 ). PCR and Sanger sequencing results also revealed the presence of another intact allele that retained the LINE/LTR elements ( Fig. 3a,b and Supplementary Figs 6a,b–12a,b ). We further demonstrated the presence of these CNAs in a portion, but not all, of the pluripotent stem cells, including ESCs, ntESCs and iPSCs, by single-cell PCR analysis ( Fig. 3c ) [52] , [53] . We conclude that the pluripotent cells are heterogeneous in terms of these repeated CNAs. Subsequently, eight single iPS cells that were randomly isolated from the 2 0 -iPSC line were cultured separately into subclonal iPS cell lines. In terms of the proportion, approximately half, of cells with deletion allele in the 2 0 -iPSC line ( Fig. 3c ), the probability function of binomial distribution determined that the eight single iPS cells, at a probability of 99%, should include at least one cell with deletions and one cell without any deletion. Surprisingly, single-cell PCR analysis also demonstrated a mixed composite of cells with and without the repeated deletions in each subclonal iPS cell line ( Supplementary Fig. 13 ). This additional experiment supports that genetic heterogeneity is a fundamental characteristic of pluripotent cells, regardless of the identity of the initial single cell. The additional differentiation experiments confirmed that the CNAs preferentially occurred in the pluripotent stem cell lines and then disappeared during the process of differentiation ( Fig. 4a and Supplementary Figs 6c–9c, 11c, 12c, 14 ). This pattern had no relationship with the cell culture passages because the CNAs were retained in distinct passages of iPSC lines but did not emerge due to extended cell culture passages in other differentiated cell lines ( Supplementary Fig. 15 ). Furthermore, we demonstrated that these CNAs could be detected in blastocysts but disappeared in the fresh tissues of adult mice with the same genetic background as iPSCs ( Fig. 4b and Supplementary Figs 6d, 7d,e, 8d, 9d–f, 10c, 11d,e, 12d ). Taken together, these data provide evidence that these CNAs are unique to pluripotent stem cells ( Fig. 4c ). Figure 3: Repeated copy-number alterations (CNAs) in pluripotent stem cells. ( a ) PCR results for the iPSC-specific CNA at chr14:75,825,104–75,831,195 (upper panel) and the control intact allele that retained the CNA (lower panel). A unique amplified breakpoint-spanning PCR product was present in all of the pluripotent stem cell lines but not in all of the somatic cell lines. ( b ) Sanger sequencing of the amplified band and schematic of the PCR validation assay design. The exact deletion breakpoints were confirmed, and the deleted regions were in accordance with the annotation of the retrotransposon (LINE). ( c ) The single-cell PCR results for all of the 12 validated CNAs (from lane 2 to lane 13 according to the chromosome position of the CNAs) in 2 0 -iPSC-32, ES-8 and NTES-1. Full size image Figure 4: Disappearance of CNAs during the in vitro differentiation of pluripotent stem cells and tissues. ( a ) PCR analysis of the gradually differentiated cells demonstrating that the validated CNA at chr14:75,825,104–75,831,195 became undetectable during the in vitro differentiation of iPSCs and ESCs (left image). The corresponding PCR results for the control are shown in the right image. ( b ) The CNA validated above could not be detected in all of the tested tissues but was detected in pre-implantation blastocysts by PCR (upper panel). A unique band retaining the LINE region was also produced by PCR (lower panel). ( c ) Summary model illustrating that the pluripotent stem cells were heterogeneous in terms of the repeated CNAs and that the CNAs were unique to pluripotent cells and subsequently disappeared in differentiating cells. Full size image In summary, our study demonstrates for the first time the impact of induced or enlarged mutations on the developmental potential of the resultant iPSCs via a sequential reprogramming system. Forty-four non-synonymous accumulated SNVs may account for the success of the sequential all-iPSC mice for up to six generations through tetraploid complementation, but the viability of the mice decreased with increasing generations. Notably, the pivotal genes ( EP300 , Ryr2 , Chd2 ) involved in heart and kidney development were found to be disrupted in later-generation iPSCs. And the corresponding histopathological examination provides good evidence that the accumulation of SNVs directly impacted the survival of later-generation all-iPSC mice. However, the exact functional effects of SNVs associated with the gradually reduced viability of all-iPSC mice must be experimentally characterized in future studies. Moreover, compared with the serial SCNT experiments, the repeated generation of pluripotent cell lines might have experienced additional stress from the in vitro cell culture, potentially resulting in an increased rate of mutations, as observed in the present study. Therefore, a joint effect of the direct reprogramming strategy and the addition of an HDAC inhibitor may eliminate cloned embryos with abnormalities and facilitate serial re-cloning of mice up to 25 generations by SCNT. Importantly, the results of our present study provide information to better understand the association between gene mutations and developmental effect, which is essential for screening pre-clinical bio-safety iPSCs. Unexpectedly, the comparison of multiple sequential profiles highlights a unique pattern of CNAs in pluripotent stem cells that were ignored in previous studies on the basis of a paired comparison [18] , [20] , [54] , [55] , [56] . Moreover, not only PCR and Sanger sequencing data but also the genomic sequencing reads do confirm the presence of the repeated CNAs in pluripotent stem cells and the disappearance of the CNAs in differentiating cells and somatic cells. These subtle genome alterations occur primarily in the retrotransposons of pluripotent stem cells, including iPSCs, ntESCs, ESCs and pre-implantation blastocysts from which ESCs are derived, suggesting a common characteristic of self-renewing pluripotent stem cells [57] . The single-cell PCR and subclonal iPSC lines analysis further indicate that the allele deletion of LINR/LTR may contribute to the heterogeneity in pluripotent stem cells. Although this experimental phenomenon is interesting, the exact explanation for why such a phenomenon occurred requires more subsequent experimentation. Previous study provided a recurrent deletion mechanism of LTR transposable elements in Drosophila due to double-strand breaks beside the retrotransposon sequence with an opening of the chromatin [58] . However, the underlying molecular mechanism of repeated LINE/LTR deletion occurring in pluripotent stem cells necessitates a more thorough investigation in the future. Animal use and care All of the animal procedures were performed according to the ethical guidelines of the National Institute of Biological Sciences, NIBS. Cell culture Mouse embryonic fibroblasts (MEFs) were derived from 13.5 days post coitum (dpc) embryos collected from female 129/Sv mice that were mated with Rosa26-M2rtTA transgenic mice. Adipocyte progenitor cells (APCs) were generated and cultured as previously described [59] . Briefly, APCs were derived from the stoma-vascular fraction from the inguinal fat deposits of 10-week-old or E19.5 all-iPSC mice. ES cells and iPS cells were cultured on mitomycin C-treated MEFs in ES medium, which contained DMEM (Gibco Invitrogen, Carlsbad, CA) supplemented with 15% FBS, 1 mM L -glutamine, 0.1 mM mercaptoethanol, 1% non-essential amino acid stock and 1,000 U ml −1 LIF (all from Chemicon, Temecula, CA). Generation of iPSCs The lentivirus-based plasmids and the procedure employed for iPS cell derivation have been previously reported [15] . The viral supernatants containing the TetO-FUW-Oct4, Sox2, Klf4 and c-Myc plasmids and the packaging plasmids ps-PAX-2 and pMD2G were harvested, and the MEFs were infected with supernatants containing viruses at a density of ~5 × 10 5 cells per 6-cm dish. The infection medium was replaced with ES medium supplemented with 1 μg ml −1 Dox 12 h after the infection. The ES-like colonies appeared after ~12 days, and, 4 days after the withdrawal of Dox, smooth colonies were isolated and passaged for an additional 3 days to derive the 1 0 - iPSC lines. APCs were retrieved from the all-iPSC mice generated from the 1 0 -iPSCs through tetraploid complementation. Under Dox induction, 2 0 -iPSCs were subsequently established. The 3 0 -iPSCs, 4 0 -iPSCs, 5 0 -iPSCs and 6 0 -iPSCs were all derived from the preceding ‘all-iPSC’ mice using the same induction method. AP and immunofluorescence staining AP staining was performed using the alkaline phosphatase detection kit (Millipore) according to the manufacturer’s instructions. Immunofluorescence staining was performed as previously described [15] . iPS cells growing on the gelatin-coated cover slides were fixed in 4% paraformaldehyde overnight at 4 °C. After permeabilization with 0.1% Triton X-100 and blocking with 2.5% bovine serum albumin for 1 h at room temperature, iPS cells were incubated with the primary antibodies to anti-Oct4 (1:500; Santa Cruz), Sox2 (1:1,000, Abcam), Nanog (1:1,000; Cosmo BioCo) and SSEA-1 (1:50; Abcam) for 2 h at room temperature separately. After three times of washing, the samples were incubated with Alexa-Fluor goat anti-rabbit or goat anti-mouse IgG secondary antibodies (1:1000; Invitrogen) for 1 h at room temperature. DNA was labelled by DAPI. Stained cells mounted on slides were observed on a LSM 510 META microscope (Zeiss) using Plan Neofluar × 63/1.4 Oil DIC objective. In vitro differentiation of iPSCs and adipogenesis The iPSCs were trypsinized and cultured in 20-μl hanging drops (1,000 cells per drop) supplemented with DMEM, 10% FBS, 1 mM L -glutamine, 0.1 mM mercaptoethanol and 1% non-essential amino acid stock without LIF. Embryoid bodies from the hanging drops were collected at 2 days and transferred to ultra-low cluster plates (Costar) for 3 days. Next, the embryonic bodies were harvested and plated onto gelatin-coated tissue culture dishes for another 15 days. Spontaneous differentiation was examined by quantitative PCR and PCR with reverse transcription for representative lineage-specific marker genes at various time points (day 2, day 4, day 6, day 10, day 20). Differentiation of the APCs into adipocytes was performed using the human mesenchymal stem cell kit (Lonza) according to the manufacturer’s instructions. Bisulfite sequencing Genomic DNA was isolated with phenol:chloroform:isoamyl alcohol (25:24:1) using a standard protocol and treated with the EpiTeck Bisulfite Kits (Qiagen). Two rounds of nested PCR was performed to amplify the promoter region of Oct4 and Nanog. The PCR products were cloned into the vector using the pEASY-T5 Zero cloning kit (TransGen Biotech), and 12 randomly selected clones were sequenced. Pluripotency validation of iPSCs iPSCs (2–5 × 10 6 ) were subcutaneously injected into the forelimb of severe combined immunodeficient mice. Four weeks after the injection, the tumours were dissected and processed for haematoxylin-eosin staining. To produce chimeric mice, 10–15 iPSCs were microinjected into eight-cell ICR embryos using a piezo-actuated microinjection pipette. After culturing for 1 day, the embryos were transplanted into the uteruses of pseudo-pregnant mice. To perform tetraploid embryo complementation, two cell-stage ICR embryos were electrofused to produce tetraploid embryos, and 10–15 iPSCs were subsequently injected into the reconstructed tetraploid blastocysts. Caesarean sections were performed at E19.5, and the pups were fostered by lactating ICR mothers. The primer sequences used for SSLP analysis were obtained from the Mouse Genome Informatics website ( http://www.informatics.jax.org ). Sample preparation and genome sequencing All of the pluripotent stem cells (sequentially iPSCs, ntESCs, ESCs) were cultured under the same standardized conditions and collected at approximately passage 10. However, R1 ESCs were cultured and collected at passage 30. The somatic cells from all-iPSC mice were cultured and collected at passage 2. After removing the feeder cells, genomic DNA was extracted from the cell pellets using the DNeasy Mini Kit (Qiagen), and the DNA was quantified using a Qubit 2.0 Fluorometer (Life Technologies). The library construction and sequencing, including five somatic cell lines and eight iPSC lines, were performed according to the standard manufacturer’s instructions for the HiSeq 2000 system. Whole-genome sequencing was applied to generate paired-end reads with a length of 101 bp. Raw reads were aligned to the mouse genome NCBI37/mm9 assembly by the Burrows–Wheeler aligner with default parameters [60] . Only uniquely mapped reads with a quality score >15 were retained for downstream analysis. For each sample, the data provided ~50-fold coverage of the mouse genome ( Supplementary Fig. 2a ). Analysis of MeDIP sequencing and RNA sequencing MeDIP-seq and RNA-seq of all eight sequential iPSC lines were conducted as previously described [24] . In brief, the genomic DNA was sonicated to 100–500 bp and adaptor was then ligated to the end of the DNA fragments according to the paired-end DNA sample prep kit (Illumina). Then the DNA was immunoprecipitated with the 5 mC antibody using the magnetic methylated DNA Immunoprecipitation kit (Diagenod). After the immunoprecipitated DNA was amplified for approximately 12–15 cycles, fragments of the proper size (200–300 bp) were gel-purified using the Gel Extraction Kit (Qiagen). The paired-end sequencing was performed at the Beijing Genomics Institute (ShenZhen, China) using the HiSeq 2000 system developed by Illumina. The MeDIP sequencing reads were aligned to mouse genome NCBI37/mm9 via using the Burrows–Wheeler aligner [60] . The uniquely aligned reads were retained and fed into MACS2 (ref. 61 ). The ‘macs2 callpeak’ command with an adjusted cut-off P value of 1−e5 was used to evaluate the DNA methylation peaks. The peak profiles of all-iPSC lines were utilized to define the DMRs across the sequential reprogramming. We further obtained the accumulating pattern of DMRs in promoter regions, (−1.5 kbp, 500 bp) around the transcription start sites (annotated in UCSC genome browser, http://genome.ucsc.edu ). Total RNA was isolated from cell pellets using TRIzol reagent (Life Technologies). The mRNA was enriched using oligo (dT) magnetic beads and sheared to create short fragments of ~200 bp. Subsequently, cDNA was synthesized using random hexamer primers and purified. Finally, the sequencing primers linked to the cDNA fragments were isolated by gel electrophoresis and enriched by PCR amplification to construct the library. Single-end sequencing was applied to the RNA sequencing. The RNA sequencing reads were aligned by TopHat with the annotation file fetched from the UCSC genome browser ( http://genome.ucsc.edu ). The FPKM for each gene was then calculated using cufflinks based on the coverage information generated from TopHat [62] , [63] . Differentially expressed genes were identified on the basis of a comprehensive consideration of the P value and fold-change via the ‘Cuffdiff’ command. Tracing SNVs during sequential reprogramming The ‘Mpileup’ command in SAMtools was used to generate the basic information for identifying variants [64] . The following criteria were applied: (1) the minimum coverage of the variant sites was 20; (2) the Phred-scaled base quality was >15; (3) the mutant allele frequency was >0.3, however, there could be no reads for the mutant allele in the control sample; and (4) the mutant allele was supported by both the forward and reverse strand reads. We collected each SNV through pair-wise comparisons and calculated the mutant allele frequency in all 13 sequential samples. The SNVs were divided into four categories on the basis of the characteristics of the allele frequencies among the 13 samples. SNV validation The single-nucleotide variants were validated via multiplexed genotyping reactions with a Sequenom MassARRAY Analyzer [65] . The primers were designed using the online genotyping design tools available in the Assay Design Suite ( https://www.mysequenom.com/Tools ). All of the experimental processes, including the PCR reactions, SAP reactions and extend reactions, were manipulated according to the standard procedures supplied by Sequenom in triplicate. Among the 20,000 mutant sites detected in the sequencing data, 189 sites were selected that were randomly distributed in the four SNV categories for validation. The mutant allele frequencies in all 13 sequential samples were verified, and the frequency in the feeder cells was also verified to exclude the effects of feeder cell contamination. Digital PCR to estimate the SNV cell frequency in somatic cells and iPSCs Digital PCR was performed as previously described using the Bio-Rad QX100 ddPCR system [47] , [48] . In our experience, for samples of this nature, the optimal concentration of genomic DNA is 24 ng per 20 μl, although a series of concentrations (3 ng per 20 μl, 12 ng per 20 μl, 24 ng per 20 μl, 48 ng per 20 μl) was tested to reduce the solution viscosity and ensure a sufficient number of droplets. For each SNV, we performed Custom TaqMan SNP Genotyping Assays (Life Technologies), which contained sequence-specific forward and reverse primers to amplify the polymorphic sequence of the SNV and two TaqMan MGB probes. One probe was labelled with VIC dye and used to detect the reference allele sequence, and another probe was labelled with FAM dye and used to detect the mutant allele sequence. TaqMan assays were conducted at a final concentration of 900 nM of each primer and 250 nM of each probe in all ddPCR reactions. According to the manufacturer’s instructions, DG8 cartridges were loaded with 20 μl PCR reaction mixtures consisting of ddPCR Supermix for the TaqMan assay, and 70 μl of droplet generator oil was used for each sample. The cartridges were placed into a droplet generator for the emulsification of 15,000–20,000 water-in-oil droplets, and the emulsified samples were transferred onto a 96-well plate. PCR was then performed using the following programme: 95 °C for 10 min, 40 cycles of 94 °C for 30 s, 60 °C for 1 min, and 98 °C for 15 min. Each chemically homogenous droplet supported PCR amplification in a thermal cycler (C1000 Touch, Bio-Rad Laboratories). Finally, the PCR products were analysed using a droplet reader (QuantaLife) to count the number of positive and negative droplets based on the fluorescence. It should be noted that the FAM-positive droplets indicated the occurrence of SNVs, and the VIC-positive droplets represented the reference base. The application of Poisson statistics allowed us to estimate the absolute number of copies of both genotypes in the cell lines. After comparing the concentrations between the mutant and wild type, the mutant allele frequency of each SNV was evaluated. Moreover, no-template controls containing TE buffer (10 mM Tris, 0.1 mM EDTA, pH 8.0) in place of DNA in the TaqMan assays were analysed to eliminate results representative of low-level template contamination. Detection of CNAs via read depth and paired-end analysis By adopting a mean-shift approach after GC correction, CNVnator was used to detect abnormal segments on read-depth ratio profiles [66] . To obtain ultra-deep coverage in our experiment, 100-bp bins were used for segmentation. The parameter ‘-relax’ was adjusted from default frequencies of 0.25 to 0.125, which made the CNVnator more sensitive for the detection of ‘gain’ or ‘loss’ segments with lower cell frequencies in pluripotent stem cells. Breakdancer, a method that is used to determine the orientation of reads and the abnormal span range of paired reads in contrast to the library insert size in library construction, was used to detect the specifically occurring CNA pattern in iPSCs [67] . A CNA that was found to be repeated in at least five iPSC lines but was not detected in any of the somatic cells was regarded as a potential CNA for further study pending validation. We manually checked the repeated CNA candidates in 13 sequential samples, allowing both ends of a CNA in multiple samples to deviate up to 50 bp due to variability in the CNA determination. PCR and Sanger sequencing for CNA validation To validate the repeated CNAs in pluripotent stem cells, we used Primer-BLAST ( www.ncbi.nlm.nih.gov/tools/primer-blast/ ) to design specific primers to amplify the breakpoint-spanning or other complex region with structural variation such as a duplication or insertion. To demonstrate the presence of an intact allele that retained the deleted region, primers were designed to target the deleted region and its adjacent areas. The optimal primers were defined to be 20–25 bp in length and had a Tm of 58–62 °C and a GC content of 45–55% to ensure the amplification of only specific PCR products in the presence of deletions or other structural variations. PCR was conducted with 20-μl reactions consisting of 10 × Ex Taq Buffer (TaKaRa), 0.1 μl TaKaRa Ex Taq HS (5 units μl −1 ), 1.6 μl dNTP mixture (2.5 mM), 0.5 μl each of forward and reverse primers at a concentration of 10 μM and ~100 ng of genomic DNA in sterilized distilled water. The reactions were performed using a thermal cycler (Bio-Rad) with the following conditions: 95 °C for 3 min, 35 cycles of 95 °C for 30 s, 58–62 °C (according to the primers), 72 °C for 30 s and a final extension of 72 °C for 5 min [47] . The CNA candidates were screened using all of the somatic cell lines and pluripotent stem cell lines. If a single amplified product was present in each pluripotent stem cell line but no somatic cell lines, the repeated CNAs were validated. These validated CNAs were subsequently analysed in gradually differentiated cells. All of the specifically amplified PCR products were purified using the QIAquick PCR Purification Kit. Sanger sequencing of the extracted DNA was performed using both forward and reverse primers. The resulting sequences were aligned to the reference genome using the online sequence alignment tool BLAT. To validate the CNAs in single cell of the 2 0 -iPSC-32, ES-8 and NTES-1 cell lines, we used the single-cell whole genome amplification kit (Yikon Genomics) to efficiently amplify genomic DNA from single cells according to the manufacturer’s instructions [52] , [53] . The products were then used as a template for PCR validation of the CNAs. Accession codes : The raw whole-genome sequencing data reported in this study have been submitted to the Sequence Read Archive (SRA) at NCBI (accession number SRP029308). How to cite this article: Gao, S. et al . Unique features of mutations revealed by sequentially reprogrammed induced pluripotent stem cells. Nat. Commun. 6:6318 doi: 10.1038/ncomms7318 (2015).